Long livestock farming history and human landscape shaping revealed by lake sediment DNA The reconstruction of human-driven, Earth-shaping dynamics is important for understanding past human/environment interactions and for helping human societies that currently face global changes. However, it is often challenging to distinguish the effects of the climate from human activities on environmental changes. Here we evaluate an approach based on DNA metabarcoding used on lake sediments to provide the first high-resolution reconstruction of plant cover and livestock farming history since the Neolithic Period. By comparing these data with a previous reconstruction of erosive event frequency, we show that the most intense erosion period was caused by deforestation and overgrazing by sheep and cowherds during the Late Iron Age and Roman Period. Tracking plants and domestic mammals using lake sediment DNA (lake sedDNA) is a new, promising method for tracing past human practices, and it provides a new outlook of the effects of anthropogenic factors on landscape-scale changes. The concept of the Anthropocene [1] recognizes that humankind has become one of the many factors capable of affecting global geological processes. However, the questions of when, where and how human societies became such a geological force remain to be resolved. Landscape shaping, which affects erosion, is most likely the oldest human-caused geological process [2] , [3] . In particular, the domestication of animals has long been a determinant of the modification of landscapes [4] . However, because changes in climate also influence landscape transformations, it is often challenging to disentangle anthropogenic effects from those of a climatic origin. Past reconstructions of landscape changes and human activities are required to meet this challenge. Currently, our knowledge of ancient societies and their effects on the environment is mainly based on sparse archaeological data as well as documentary and natural archives [5] , [6] , [7] , [8] , [9] , [10] , [11] , [12] , [13] . Even recently developed proxies of pasturing activities (for example, those utilizing faecal molecules and coprophilous fungi spores in lake sediments) are indirect and not specific to particular domestic animal species [5] , [6] , [7] . Thus, information available on the nature of past human activities is scattered or imprecise. It is therefore necessary to address this methodological gap to better understand the impact of human activities on local-to-global geological processes. Recent developments in the combined use of high-throughput sequencing [14] and metabarcoding approaches enable the assessment of the biodiversity of current ecosystems using extracellular DNA that is contained in environmental samples [15] , [16] . DNA from a variety of taxa, including faecal bacteria, plants and domestic mammals, has been successfully extracted and sequenced directly from natural archives (frozen soils, cave sediments and lake sediments), even in the absence of visible macrofossils [17] , [18] , [19] , [20] , [21] , [22] , [23] , [24] , [25] . The application of DNA metabarcoding to lake sediments has also proven its potential to trace past vegetation cover [22] . However, this tool has never been used with the objective of detecting the presence of mammals and plants in ancient ecosystems and to reconstruct a detailed picture of human land use since the Neolithic Period. Here we test whether the application of the metabarcoding approach to high-resolution lake sediment archives can provide reliable and novel information regarding human occupation. We use the well-described sediments of the subalpine Lake Anterne [26] , which is located in the North French Alps (2,063–2,478 m asl) above the present treeline ecotone ( Fig. 1 ). The catchment area of Lake Anterne has steep slopes made of calcshales and black shales, which are easily erodible rocks (see Methods). Thus, Lake Anterne sediments provide a good record of erosional processes ( Fig. 1d ). We combine results from the metabarcoding approach with a previous reconstruction of the frequency of erosive events [26] to document the effects of human activities on erosion dynamics. In particular, we investigate the hypothesis of an anthropogenic origin of the strong increase in erosion that occurred during the Roman Period, which is a supposed warm and dry climatic period [27] , expected to correspond to unfavourable conditions for erosion. Our reconstruction of the livestock farming history shows periods of grazing activity with sheep and/or cowherds that mainly occurred at the end of the Iron Age, the Roman Period, the Medieval times and the Modern Period. During the Roman Period, deforestation strongly affected Alnus sp. and the frequency of erosive events is the highest of the last 10,000 years. Together, these results suggest that the most intense grazing pressure on landscape and the erosion in this subalpine area occurred during the Roman occupation. 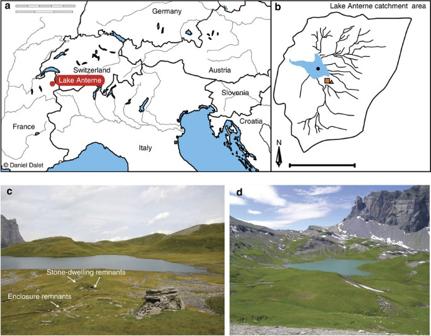Figure 1: Location and presentation of the study area. Presentations of the location of Lake Anterne (a, the upper scale bar label is 100 km and the lower is 60 mi), and of the catchment area (b, the scale bar label is 1 km) with the lake coring site represented by the black dot and the archaeological remains represented by a red square (stone-dwelling remnants) and triangle (enclosure). The Lake Anterne catchment area is 2.55 km2, the lake area is 0.12 km2and the deeper depth is 13.2 m. Panelcpresents a picture of the locations of the archaeological remains and panelda picture of the lake catchment that shows its sensitivity to erosion processes. Figure 1: Location and presentation of the study area. Presentations of the location of Lake Anterne ( a , the upper scale bar label is 100 km and the lower is 60 mi), and of the catchment area ( b , the scale bar label is 1 km) with the lake coring site represented by the black dot and the archaeological remains represented by a red square (stone-dwelling remnants) and triangle (enclosure). The Lake Anterne catchment area is 2.55 km 2 , the lake area is 0.12 km 2 and the deeper depth is 13.2 m. Panel c presents a picture of the locations of the archaeological remains and panel d a picture of the lake catchment that shows its sensitivity to erosion processes. Full size image Plant DNA and landscape changes For the first run, which included nine samples, we obtained 3,151,601 reads that represented 68,137 unique sequences. After the different filtering steps, as described in the Methods, the number of sequences was reduced to 2,140,829 (428 unique sequences). For the second run, which included 35 samples, 5,575,081 reads (386,880 unique sequences) were obtained after high-throughput sequencing. This number was further reduced to 4,059,103 after filtering (909 unique sequences). Plant contaminations, mainly from a plant sequence from the Lamiales order (42% of total read numbers after filtering), were detected in the control samples of the second run. Overall, a large dataset of plant taxa is obtained. For this study, we focused on Pinus sp. and Alnus sp. ( Supplementary Tables 1,2 ; Fig. 2 ) to document deforestation dynamics in relation to pasturing practices. 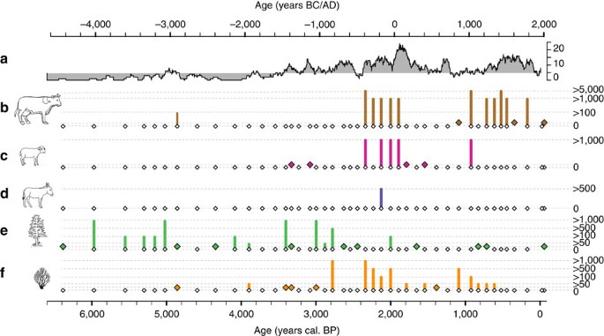Figure 2: Erosion and DNA from mammals and plants recorded in Lake Anterne sediments. The erosion signal (a) is represented by the frequency of erosive events (number of events every 100 years). This signal is compared with mammal DNA (b:Bossp. DNA,c:Ovissp. DNA,d:Equussp. DNA) and plant DNA (e:Pinussp. DNA;f:Alnussp. DNA) from lake sediments. Diamonds represent sediment samples that were taken in cores for metabarcoding analyis. Open diamonds show samples where no DNA sequences were found. Coloured diamonds show DNA sequences that were present in only one replicate. Bars reflect DNA sequences that were present in at least two replicates. The heights of the bars correspond to the ranges of the sequence numbers (that is, between 50 and 100; between 100 and 500; between 500 and 1,000; between 1,000 and 5,000; and more than 5,000). Only insignificant contaminations (one read) were observed regarding these plant taxa of interest ( Supplementary Table 2 ). Pinus sp. DNA was mainly present before 2,800 cal. yr BP. More precisely, three phases of high DNA content were recorded as follows ( Fig. 2 ): between 6,000 and 5,000 cal. yr BP; at 3,400 cal. yr BP; and between 3,000 and 2,800 cal. yr BP. High occurrences of Alnus sp. DNA were recorded after the decline of Pinus sp. DNA at 2,800 cal. yr BP, between 2,350 and 2,000 cal. yr BP and at ~1,000 cal. yr BP. Figure 2: Erosion and DNA from mammals and plants recorded in Lake Anterne sediments. The erosion signal ( a ) is represented by the frequency of erosive events (number of events every 100 years). This signal is compared with mammal DNA ( b : Bos sp. DNA, c : Ovis sp. DNA, d : Equus sp. DNA) and plant DNA ( e : Pinus sp. DNA; f : Alnus sp. DNA) from lake sediments. Diamonds represent sediment samples that were taken in cores for metabarcoding analyis. Open diamonds show samples where no DNA sequences were found. Coloured diamonds show DNA sequences that were present in only one replicate. Bars reflect DNA sequences that were present in at least two replicates. The heights of the bars correspond to the ranges of the sequence numbers (that is, between 50 and 100; between 100 and 500; between 500 and 1,000; between 1,000 and 5,000; and more than 5,000). Full size image Mammal DNA and livestock farming history For the first and second runs, we obtained 967,653 and 1,029,717 reads, respectively, after high-throughput sequencing (81,011 and 81,684 unique sequences, respectively). After filtering, the number of sequences was reduced to 165,373 (19 unique sequences) for the first run and 78,910 (29 unique sequences) for the second run. For this study, three mammalian genera that are known to be associated with human activities were selected ( Supplementary Tables 1,2 ; Fig. 2 ): Bos sp., Ovis sp. and Equus sp. Only insignificant contaminations (one or two reads) were observed regarding these genera ( Supplementary Table 2 ). Cow DNA was detected in at least two PCRs during the Neolithic Period (4,800 cal. yr BP), at the end of the Iron Age/onset of the Roman Period (2,400–1,900 cal. yr BP) and during the Medieval-Modern times (~1,000 AD; between 1,200 and 1,500 AD; and at 1,750 AD). In at least two PCRs, sheep DNA was found at the end of the Iron Age/onset of the Roman Period and at ~1,000 AD. Equus sp. DNA was also recorded at 2,100 cal. yr BP. Over the last 6,500 years, the highest cow and sheep DNA contents were observed at the end of the Iron Age, onset of the Roman Period and the Medieval-Modern times ( Supplementary Table 2 ). In this study, we evaluated whether DNA metabarcoding applied to lake sediment was a reliable approach for tracing the history of human activities and landscape changes. In practice, the reliability of the lake sediment DNA (sedDNA) record can be affected by taphonomical processes, which implicate several factors. First, physicochemical conditions and sediment composition must be favourable to avoid the complete degradation of DNA. In Lake Anterne, sediment compounds, such as clays, sands, humic substances and organomineral complexes, that allow DNA adsorbance, together with cold temperature and periodic anoxic conditions on the lake bottom (see Methods), are likely to have favoured DNA preservation [28] , [29] , [30] . Moreover, DNA was present in all samples, even the oldest, suggesting that the DNA was sufficiently preserved to successfully reconstruct the presence of the taxa of interest. Second, DNA mixing through water circulation in lake sediment layers must be a minor process to maintain the DNA stratigraphic position. Lake sediments are permanently saturated with water, which prevents percolation of liquids and, thus, DNA leaching. Before sediment compaction, vertical advection of pore water can occur within the first centimeters at the water/sediment interface. However, in the case of Lake Anterne, the sediments are mainly clastics, which induce fast compaction and limit the thickness where mixing is possible. After compaction, vertical advection becomes minimal [19] , [22] . Thus, we assume that the temporal succession of our DNA record was not disturbed. The reliability of a lake sedDNA record also depends on potential bias linked to the analytical techniques (possible contamination, amplification and sequencing errors). However, strict precautions were taken in the laboratory at each step of the experiment to avoid contamination. All the laboratory steps (sediment core sampling, DNA extraction and DNA amplification) were performed in a room where no DNA research had previously been performed and in rooms that were specifically dedicated to ancient DNA. In addition, replicates during the sampling, extraction and amplification steps allowed an optimal chance to obtain mammal and plant DNA sequences and enabled us to detect sporadic contamination, which is expected to be present in only one of eight replicates. Appropriate data treatment was also performed to filter out amplification and/or sequencing errors. These measures and the quasi-absence of contamination in the negative controls confirmed the quality of our data. Moreover, the temporal consistency of the plant and mammal DNA analyses (no random distribution of the data) further strengthens the confidence in our lake sedDNA data. Finally, other results from independent archives and proxies provided an independent validation of a portion of our lake sedDNA results. Indeed, the pattern of tree cover that was revealed by our lake sedDNA is concordant with previous regional palynological studies that were performed near the Anterne catchment (Sur Villy, 2,235 m asl; Ecuelles, 1,850 m asl) [31] , [32] . Moreover, in support of the reconstruction of livestock farming that was obtained using mammal DNA, one enclosure and two stone-dwelling remnants were found near the lake ( Fig. 1b,c and Supplementary Fig. 1 ). The foundation of the dwelling closest to the lake was dated to the Second Iron Age (2,335–2,155 cal. yr BP), but, according to ceramic analysis (unpublished data) and 14 C dating on charcoal (1,865–1,705 cal. yr BP), the most intense occupation most likely occurred at the beginning of the Roman Period. One hundred and fifty-two bone remains that were found at the site were determined (unpublished data) as follows: one hundred and forty-three were attributed to sheep ( Ovis aries ) or goat ( Capra hircus ), six were attributed to sheep and three were attributed to domestic rooster ( Gallus gallus domesticus ). The presence of these bones allowed, at least in part, for the validation of our mammal DNA results. The lack of cattle bones may have occurred because these animals were not eaten on site or because of the limited archaeological research in this zone. The transition at ~1,200 AD from a mix of sheep and cowherds to a dominance of cowherds has been previously documented through historical archives [5] , [33] of the same period (between 1,300 and 1,500 AD) in the French and Swiss Alps, which again validates our DNA results. However, our study is the first to track such land-use changes using a natural archive. This approach enabled a more precise detection of past land-use practices, especially for prehistoric periods and locations where no written traces were left by inhabitants. We did not record sheep DNA in the lake sediments that corresponded to the present day, although we have evidence of the presence of sheep at a low density in the catchment periodically during the summer. This result highlights the need of a relatively high amount of mammalian DNA that was transferred to the lake to be detected in the sediments (see Supplementary Discussion about mammalian DNA detection) and shows that the absence of DNA in lake sediments should be treated with caution, as this does not necessarily highlight the absence of the targeted species. In contrast, no cattle herd is currently in the catchment, but we record the presence of cow DNA in one of eight PCRs of the recent lake sediments, which may be explained by sporadic contamination or stocking of older cow DNA in soils because it is known that DNA can persist in alpine soils for at least 50 years [34] . Thus, these results, which are contradictory to expectations, reveal that lake sedDNA allows the reconstruction of past livestock history with a high level of confidence when the stocking rate (in animal unit per day ha −1 ) is relatively high and/or the practice induces important transfer of domestic mammal DNA (mainly from faeces, skin flakes and chitinous material [35] ) to the lake. On the basis of these considerations, the main phases of livestock farming in the subalpine Lake Anterne catchment occurred during the end of the Iron Age, the Roman Period and the Medieval-Modern times. The second objective of our study was to integrate our lake sedDNA record in the context of the erosion dynamic history to bring a novel perspective regarding human/environment interactions, in particular during the Roman Period (0–200 AD), which was when the highest frequency of erosive events of the entire Holocene Period was recorded [26] ( Fig. 3 ). As shown by the reconstruction of Aletsch glacier fluctuations (Swiss Alps), the Roman Period was characterized by a warm and/or dry climate [27] ( Fig. 3 ), that is, conditions that are not favourable to erosion. On the basis of these facts, we previously hypothesized that human-associated activities were the primary determinants of the increased frequency of erosive events [36] during this period at Lake Anterne. Our lake sedDNA record ( Figs 2 , 3 ) provides new evidence to support the ‘human impact’ hypothesis of this erosion paroxysmal phase, and provides a more comprehensive picture regarding the nature and intensity of human practices during this period. The presence of cattle and sheep DNA in lake sediments is indicative of intense pasturing activity with mixed herds in the catchment. Grazing has strong effects on soil erosion through direct processes, such as soil compaction, reduction of infiltration and detachment of particles, as well as indirect processes, such as the reduction of vegetation cover and development of bare and unstable soils [37] . The disappearance of Alnus sp. ( Fig. 2 ) may reflect subalpine forest clearance, and this change in the landscape vegetation suggests significant grazing pressure that was most likely associated with a high stocking rate. The direct effects of trampling and grazing by herds, as well as the drastic reduction of the tree cover on soil stability, help to explain the extensive erosion that was recorded in lake sediments of this period. 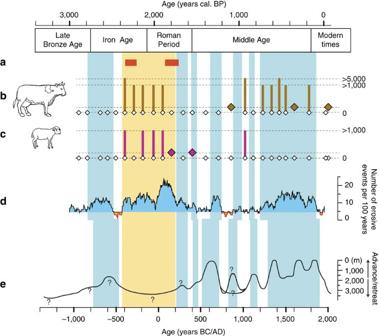Figure 3: Effects of pasturing activity and climate on erosion over 3,000 years. We present a comparison between data about human occupation and activities from the archaeological survey (a: red squares representing charcoal dating from the stone-dwelling remnants), lake sediment DNA (b:Bossp. DNA,c:Ovissp. DNA), the reconstruction of local erosion dynamic (d: Lake Anterne erosion indicator) and a proxy of climatic conditions in the western part of the Alps (e: Aletsch Glacier fluctuations27). The question marks on the curve mean that the reconstruction of the position of the glacier terminal point is uncertain. Diamonds represent sediment samples that were taken in cores for metabarcoding analyis. Open diamonds show samples where no DNA sequences were found. Coloured diamonds show DNA sequences that were present in only one replicate. Bars reflect DNA sequences that were present in at least two replicates. The heights of the bars correspond to the ranges of the sequence numbers (that is, between 50 and 100; between 100 and 500; between 500 and 1,000; between 1,000 and 5,000; and more than 5,000). The orange coloured area represents the period of glacier retreat (warm and/or dry period) that was associated with high erosion. The blue coloured areas represent the period of glacier advances (cold and/or wet periods) that were associated with high erosion. Figure 3: Effects of pasturing activity and climate on erosion over 3,000 years. We present a comparison between data about human occupation and activities from the archaeological survey ( a : red squares representing charcoal dating from the stone-dwelling remnants), lake sediment DNA ( b : Bos sp. DNA, c : Ovis sp. DNA), the reconstruction of local erosion dynamic ( d : Lake Anterne erosion indicator) and a proxy of climatic conditions in the western part of the Alps ( e : Aletsch Glacier fluctuations [27] ). The question marks on the curve mean that the reconstruction of the position of the glacier terminal point is uncertain. Diamonds represent sediment samples that were taken in cores for metabarcoding analyis. Open diamonds show samples where no DNA sequences were found. Coloured diamonds show DNA sequences that were present in only one replicate. Bars reflect DNA sequences that were present in at least two replicates. The heights of the bars correspond to the ranges of the sequence numbers (that is, between 50 and 100; between 100 and 500; between 500 and 1,000; between 1,000 and 5,000; and more than 5,000). The orange coloured area represents the period of glacier retreat (warm and/or dry period) that was associated with high erosion. The blue coloured areas represent the period of glacier advances (cold and/or wet periods) that were associated with high erosion. Full size image ‘Natural History’, written by Pliny the Elder in 77–79 AD, describes the manufacturing of one of the most popular cheeses in Rome, which was made from cow milk in the Centronian Alps (corresponds approximately to the North French Alps) (see Supplementary Note 1 ). Pliny’s statement suggests the development of a pastoral activity that was profitable enough to engage in an important cheese trade with Rome, which was ~1,000 km away. The high amount (high number of reads in two of eight replicates; Supplementary Table 2 ) of cattle DNA in the sedimentary record is consistent with a boom in this type of economy. The temporal depth of our natural archive shows that this activity most likely began at the end of the Iron Age (400 BC) ( Fig. 3 ) and, thus, occurred before the Roman invasion of the region in 76 BC. Furthermore, the presence of equine DNA at 200 BC ( Fig. 2 ) suggests that intensive farming activities had already been organized by the Gallic people in this high-altitude pasture. Nevertheless, because we recorded an expansion of Alnus sp. and a lower increase in the frequency of erosive events than during the Roman Period, grazing pressure and, consequently, farming activity were most likely less important ( Fig. 2 ). The Roman intensification of livestock farming, which required more space for grazing, most likely explains the complete disappearance of Alnus sp [31] , [32] . ( Fig. 2 ). Finally, at the end of the Iron Age, the green alder shrub expansion, which stabilized the soil cover, and the dry climatic conditions [27] , [36] supported a major role of sheep and cowherds in catchment erosion. The metabarcoding approach applied on lake sediments reveals valuable and novel data on the occupation dynamics of the European Alps, as it provided the first high-resolution reconstructed history of livestock farming over six millennia at the species level. Nevertheless, independent and complementary data (sedimentological, palynological, archaeological and historical) are certainly important when validating and interpreting lake sedDNA analyses. By combining sedimentological data and lake sedDNA evidence, we showed that overgrazing by sheep and cowherds associated with deforestation triggered the most important erosion crisis of the Holocene in the Anterne catchment, which occurred during the Roman Period. Finally, we provided evidence for an important role of livestock farming on erosion dynamics, which allowed for the discrimination of the effects of climate and anthropogenic drivers. SedDNA would be of great interest to the archaeological and anthropological communities. In addition to classical palaeoenvironmental approaches, the use of lake sedDNA will likely become a new approach for reconstructing Holocene palaeoenvironments to better understand the human/climate/environment interactions during the Anthropocene. Study site Lake Anterne is a high-altitude lake (2,063 m asl, 0.12 km 2 and 13.2 m maximum water depth) that is located in the Northern French Alps ( Fig. 1a,b ). Lake Anterne has a small catchment (2.55 km 2 ) with steep slopes that are composed of easily erodible rocks (calcshales, namely, Bajocian; and black shales, namely, Bathonian–Oxfordian). The following three main soil types were identified in these rocks: leptosols (~50% of the catchment area), cambisols (~25%) and acid soils (podzosols/stagnosols; ~15%) [26] . These soil types represent different stages of soil development (from less- to more-developed soils). Given the presence of easily erodible material on steep slopes, the lake sedimentation is mainly due to erosion processes ( Fig. 1d ). This sedimentation consists of clastic laminations that were formed by erosive events (mainly floods triggered by precipitation events) [33] . The lake is frozen 6–7 months per year, which favours anoxic conditions at the lake bottom. During summer, anoxic conditions also occur periodically (Giguet-Covex unpublished data) and are most likely due to organic matter decomposition by aerobic bacteria. During the year, the temperature at the lake bottom varies between 4 and 8 °C (Giguet-Covex unpublished data). These anoxic conditions and the low mean annual temperature favour DNA preservation [30] . A 20-m-long composite core (ANT-07) was retrieved in September 2007 from the deepest part of the lake and far from active deltas to obtain a continuous sequence that was as long as possible ( Fig. 1b ). This core, which was used for DNA analyses, was shrink wrapped to limit oxidation of the sediments and stored in a refrigerated area (4 °C; similar temperature as the lake bottom). A total of 10,160 years of environmental history could be reconstructed from this core [26] . For the present study, we focused on the last 6,400 years (16.4 m of the sediment core), which represents the period that recorded the main changes in erosion patterns [26] . Dating of the sediment core The age–depth model was based on 18 14 C measurements on terrestrial macroremains. Accelerator mass spectrometry 14 C analyses were performed by the Poznan Radiocarbon Laboratory and the LMC14 Laboratory (CNRS). All dates were calibrated (2 sigma) using the Radiocarbon Calibration Program REV 6.0.1 (ref. 38 ) and Intcal09 calibration curve [39] ( Supplementary Table 3 ). The age–depth model was then constructed without taking into account instantaneous deposits (thicker than 5 mm) [26] and by fitting a cubic spline curve using the MCAgeDepth software [40] ( Supplementary Fig. 2 ). Frequency of erosive events To determine the frequency of erosive events, the sedimentary deposits that resulted from these events were visually identified and documented in terms of stratigraphic location. Visual identification was based on the sedimentological features of these deposits. These features are characterized by the succession of three phases that become finer upward [36] , [41] from bottom to top as follows: coarse and well-sorted sediments; a mixture of silts and fine sands; and a layer of fine silts and clays. The thickness of these erosive deposits varies from 0.5 to 27 cm. The frequency was then computed as a running sum over a 100-year time window, as estimated by our age–depth model that was based on 14 C dating [26] . Sediment core sampling and DNA extraction Metabarcoding was performed on samples from a 16.4-m-long sediment core (ANT-07) that corresponded to the most recent 6,400 years. Sediment core sampling was performed in an isolated laboratory at Université de Savoie, where no DNA research had previously been performed (as suggested in Cooper and Poinar [42] ). Forty-four slices were sampled from the core, and the edges of the slices were removed to avoid contamination from water spreading along the core. Each sample was divided into two subsamples. The weight of the sediment that was obtained and used for extractions was 13.71±1.15 g. Two DNA extractions were performed per subsample (that is, four extractions per sediment slice), and two PCRs were performed per extraction (that is, eight PCRs per sediment slice). This strategy allowed for the detection of possible sporadic contamination [42] . The presence of a DNA sequence in only one PCR could be due to sporadic contamination, PCR bias or stochasticity due to low DNA concentration. Four extraction controls were also processed. Each of the controls was amplified two times with the primer pairs that were used in this study (see below). These controls allow potential contaminations to be identified in the PCR products. Extracellular DNA extraction and amplification were performed in two rooms that were specifically dedicated to ancient DNA at the Laboratory of Alpine Ecology (Université de Grenoble, France). The extraction of this DNA from the core subsamples was performed by mixing the sediment with 15 ml of saturated phosphate buffer (0.12 M Na 2 HPO 4 ; pH≈8) for 15 min to release the DNA bound to particles, and the mixture was then centrifuged (10 min at 10,000 g ). The resulting supernatant was recovered and used as starting material in the extraction steps that were carried out using a commercial kit (NucleoSpin Soil; Macherey-Nagel, Düren, Germany) by skipping the lysis step and following the manufacturer’s instructions [16] . The DNA extract was eluted in 100 μl of SE buffer. DNA amplification and high-throughput sequencing We targeted two taxonomic groups as follows: mammals and plants. Mammalian DNA was amplified using a new primer pair (MamP007F, 5′-CGAGAAGACCCTATGGAGCT-3′; MamP007R, 5′-CCGAGGTCRCCCCAACC-3′), which led to the amplification of a 60- to 84-bp fragment of the mitochondrial 16S gene. These primers were designed using the ecoPrimers program [43] ( http://www.grenoble.prabi.fr/trac/ecoPrimers ). Plant DNA was amplified using universal primers ( g , 5′-GGGCAATCCTGAGCCAA-3′; and h , 5′-CCATTGAGTCTCTGCACCTATC-3′) that targeted the P6 loop region of the chloroplast trnL (UAA) intron [44] . The length of the amplified fragment is highly variable among species and ranges from 10 to 146 bp (mean length of 45 bp). To assign sequence reads to the relevant sample after high-throughput sequencing, 8-bp tags (with at least five differences between each) were added to the 5′ end of each primer [15] , [45] . All DNA amplifications were carried out in a final volume of 30 μl containing 2 μl of DNA extract. The amplification mixture contained 1 U of AmpliTaq Gold DNA polymerase (Applied Biosystems), 15 mM Tris–HCl, 50 mM KCl, 2 mM MgCl 2 , 0.2 mM of each dNTP, 0.1 μM of each primer and 4.8 μg of bovine serum albumin (BSA, Roche Diagnostic). To restrict the amplification of human DNA when amplifying mammalian DNA [46] , we designed a human-specific, blocking oligonucleotide (MamP007_B_Hum1, 5′-GGAGCTTTAATTTATTAATGCAAACAGTACCC3-3′) and added it to the PCR mixture at a concentration of 2 μM. For both primer pairs, the PCR mixture was denatured at 95 °C for 10 min, followed by 45 cycles of 30 s at 95 °C and 30 s at 50 °C (no elongation step). The PCR products were then purified and mixed together (equivolume mixes) before sequencing, which was performed using an Illumina HiSeq 2000 platform (2 × 100-bp, paired-end reads). Two different runs were performed as follows: the first run included 9 samples (called ‘RTM’) to test the method; and the second run included 35 samples (called ‘ANT’) to improve the resolution of our record. This second run also integrated the control samples. Sequence analysis and taxa assignment Sequence data were analysed using the OBITOOLS software ( http://www.grenoble.prabi.fr/trac/OBITools ). First, the direct and reverse reads that corresponded to the same DNA fragment were aligned and merged using the SolexaPairEnd program, with the quality being taken into account when merging the two reads. The ngsfilter program was then used to assign sequences to the relevant sample based on the associated primers and tags. Only sequences containing perfect tags and primers with a maximum of three errors were considered. We used the obiuniq program to merge strictly identical sequences and kept the information about the original samples they originated from. Then, the sequences were filtered using the obigrep program according to their length as follows: sequences shorter than 50 bp for the MamP007 and 10 bp for the gh primers were removed; and sequences that had an occurrence lower than 100 over the entire dataset were removed. Because we used short markers, clustering sequences at a high level of similarity, as is usually performed with this type of data [47] , was not suitable because a single difference in the nucleotide sequence often indicated different species. The obiclean program [48] was developed to detect artifactual sequences that contained amplification and/or sequencing errors. For each PCR product, the program creates networks that connect sequences with one indel or substitution difference. Two sequences are linked if the occurrence of the less-frequent sequence is less than 20% of that of the other sequence. A status is then assigned to each sequence as follows: ‘head’ (most common sequence of a network), ‘singleton’ (sequence without a variant) or ‘internal’ (sequences that are neither ‘head’ nor ‘singleton’ and that most likely correspond to amplification or sequencing errors). Only sequences that were more often ‘head’ or ‘singleton’ than ‘internal’ in the global dataset were kept for the following steps. Finally, the sequences were assigned to the relevant taxa using the ecoTag program, which finds highly similar sequences in a suitable database (created by in silico PCR from Genbank with the ecoPCR program [49] ) . Each sequence was then assigned to unique taxa. If no complete match between a unique sequence in the database and the query sequence was found, the allotted taxa corresponded to the last common node in the NCBI taxonomic tree of all the taxids that annotated the sequences and matched the query sequence [50] . Only sequences corresponding to the Viridiplantae phylum when using plant primers and to the Mammalia class when using the mammalian primers were saved for the following steps. Another filtering step was performed to disentangle sequences that were genuinely released by organisms from the lake catchment from potential sporadic contamination. A sequence was considered genuine (with a high confidence level) at a given time if it was found at least two times among the eight PCR replicates and with a minimum of five read numbers. This criterion obviously dismissed many putative taxa that were present at low abundance or had heterogeneous distribution [17] , which is why sequences that were retrieved in one replicate were represented as ‘sequences potentially present’. Accession codes: Sequences for plant and mammal DNA have been deposited in the DRYAD database under accession number http://doi.org/10.5061/dryad.h11h7 . How to cite this article: Giguet-Covex, C. et al. Long livestock farming history and human landscape shaping revealed by lake sediment DNA. Nat. Commun. 5:3211 doi: 10.1038/ncomms4211 (2014).